Strong interaction between interlayer excitons and correlated electrons in WSe2/WS2moiré superlattice 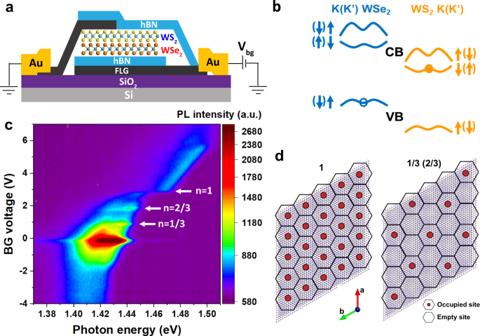Fig. 1: Interlayer exciton PL revealing correlated states in angle-aligned WSe2/WS2heterobilayer. aSchematic of the hBN encapsulated WS2/WSe2heterobilayer. One piece of few-layer graphene (FLG) is used as the contact electrode and another piece is used as the back-gate electrode with the hBN layer working as the gate dielectric.bSchematic of the type-II alignment of the WS2/WSe2heterobilayer moiré superlattice.cGate-dependent PL spectra of device D1 at 4.2 K, with CW excitation centered at 1.959 eV with an excitation power of 5 µW.dSchematics of electron (red dot) configuration for fillings ofn= 1 andn= 1/3 (2/3 and 1/3 are particle-hole symmetric) in the moiré superlattice. Heterobilayers of transition metal dichalcogenides (TMDCs) can form a moiré superlattice with flat minibands, which enables strong electron interaction and leads to various fascinating correlated states. These heterobilayers also host interlayer excitons in a type-II band alignment, in which optically excited electrons and holes reside on different layers but remain bound by the Coulomb interaction. Here we explore the unique setting of interlayer excitons interacting with strongly correlated electrons, and we show that the photoluminescence (PL) of interlayer excitons sensitively signals the onset of various correlated insulating states as the band filling is varied. When the system is in one of such states, the PL of interlayer excitons is relatively amplified at increased optical excitation power due to reduced mobility, and the valley polarization of interlayer excitons is enhanced. The moiré superlattice of the TMDC heterobilayer presents an exciting platform to engineer interlayer excitons through the periodic correlated electron states. Bilayers of two-dimensional materials with a small twist angle or a lattice mismatch can form moiré superlattices [1] , [2] , [3] , [4] , [5] . Twisted bilayer graphene at the magic angle possess flat minibands that result in strong electron interactions, enabling rich, correlated states, such as Mott insulators, unconventional superconductivity, and Chern insulators [6] , [7] , [8] , [9] . 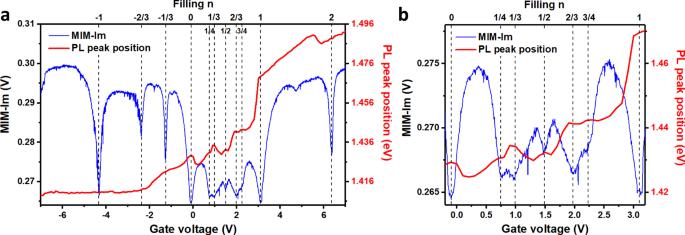Fig. 2: Identification of correlated insulating states at different fillings. aPL peak position (red) extracted from Fig.1cas a function of the gate voltage, correlated with MIM measurements of the local conductivity (blue) taken at 14 K. Dashed lines are fillings corresponding to the insulating states determined from the MIM measurements.bZoom-in of the traces from −0.2 V to 3.2 V ina. The moiré superlattice of the twisted bilayer transitional metal dichalcogenides (TMDCs) can form flat minibands with less stringent requirements, with no magic angle required. In addition, due to the large effective mass [10] , [11] , [12] , the kinetic energy is further reduced in twisted bilayer TMDCs [13] . The resulting enhanced Coulomb interaction with respect to the kinetic energy leads to strong interactions that give rise to various exotic correlated insulating states [13] , [14] , [15] , [16] , [17] , [18] , [19] , [20] , [21] with high transition temperatures. Very recently, Mott insulator states at fillings n = ±1 (one electron or hole per Moiré cell), generalized Wigner crystal states at filings n = ±1/3, ±2/3, and even more exotic insulating states at other fractional fillings have been reported [14] , [15] , [16] , [17] , [18] , [19] , [20] , [21] . The TMDCs moiré superlattice provides an exciting platform to investigate strongly correlated physics. Meanwhile, stacking two different TMDC monolayers also enables the possibility for band engineering in the heterobilayer [22] , [23] . For example, a type-II alignment in the heterobilayer allows the formation of interlayer excitons, in which the optically excited electrons reside in one layer, while the holes reside in the other layer [2] , [4] , [24] , [25] . Due to their long lifetime, valley degree of freedom, and tunability, interlayer excitons are a promising candidate for quantum emitters [3] . Both interlayer excitons and correlated electrons are results of strong interactions, and it is natural to raise the intriguing question of how they interact with each other, which, to our best knowledge, remains an uncharted territory. In this work, we explore the interaction of interlayer excitons with the correlated states in angle-aligned WS 2 /WSe 2 moiré superlattice. We find that this interaction significantly modifies the photoluminescence (PL) of the interlayer exciton. Sensitive to the change in dielectric constant and the gap opening at the correlated insulating states, the interlayer exciton PL peak energy unravels the Mott insulator state at n = 1, the generalized Wigner crystal states at n = 1/3 and 2/3, as well as at n = 1/4 and 3/4 with an even longer range interaction, and a stripe phase state at n = 1/2. Interestingly, the presence of the correlated states also significantly modifies the PL intensity. At increased optical excitation power, the PL intensity of interlayer excitons brightens up at the correlated electron states, suggesting reduced mobility of interlayer excitons in the moiré cell due to their attractive interaction with the localized correlated electrons. Furthermore, the valley polarization of interlayer excitons is strongly enhanced at certain fillings. Our results inspire engineering interlayer excitons as quantum emitter arrays through moiré potential and long-range interactions, utilizing their interplay with the localized correlated electrons. Correlated states in WSe 2 /WS 2 heterostructure The structure of our angle-aligned WS 2 /WSe 2 heterobilayer device is schematically shown in Fig. 1a . Due to the ~4% lattice mismatch, the angle-aligned WS 2 /WSe 2 bilayer would form a triangular moiré superlattice with a period of ~8 nm. The strong moiré coupling [1] , [5] will result in mini flatbands [26] , which could host correlated insulating state at half band filling with one carrier localized in one moiré cell ( n = ±1) [14] , [15] , or even at various fractional fillings of the moiré unit cell that have been interpreted as generalized Wigner crystal states [14] , [18] , [19] or stripe phases [18] , [19] , [20] . The filling patterns for n = 1 and 1/3 are shown schematically in Fig. 1d . These correlated states arise from the strong interaction between carriers, which localizes them in the moiré cells, and the formation of periodic filling pattern minimizes the overall interaction energy. Meanwhile, the energy bands of WS 2 and WSe 2 have a type-II alignment in their heterobilayer (Fig. 1b ), in which the optically excited electron will reside in monolayer WS 2 and the corresponding hole will reside in the WSe 2 layer. Due to the strong Coulomb interaction, the electron–hole pair remain bound as the interlayer exciton. Fig. 1: Interlayer exciton PL revealing correlated states in angle-aligned WSe 2 /WS 2 heterobilayer. a Schematic of the hBN encapsulated WS 2 /WSe 2 heterobilayer. One piece of few-layer graphene (FLG) is used as the contact electrode and another piece is used as the back-gate electrode with the hBN layer working as the gate dielectric. b Schematic of the type-II alignment of the WS 2 /WSe 2 heterobilayer moiré superlattice. c Gate-dependent PL spectra of device D1 at 4.2 K, with CW excitation centered at 1.959 eV with an excitation power of 5 µW. d Schematics of electron (red dot) configuration for fillings of n = 1 and n = 1/3 (2/3 and 1/3 are particle-hole symmetric) in the moiré superlattice. Full size image In Fig. 1c , we show the color plot of PL intensity as a function of photon energy and gate voltage at 4.2 K, for the interlayer exciton whose emission energy is around 1.4 eV, excited by a continuous wave (CW) laser centered at 1.959 eV with an excitation power of 5 µW. The most noticeable feature is the large energy blueshift (~20 meV) at gate voltage ~2.9 V, when the Mott insulator at n = 1 (one electron per moiré cell) is formed, as confirmed by gate-dependent reflectance spectra (see Supplementary Note 2 for details) and local conductivity measurements (Fig. 2a, b ). The relatively enhanced PL intensity at the gate voltage of ~0.9 V and ~1.9 V reveals the generalized Wigner crystal states at n = 1/3 and 2/3 (Fig. 2a, b ), respectively, likely due to the suppressed nonradiative channels at the correlated insulating states. A closer look of Fig. 1c could even resolve the states corresponding to n = 1/4 and 3/4 (see Supplementary Fig. 2 ). Fig. 2: Identification of correlated insulating states at different fillings. a PL peak position (red) extracted from Fig. 1c as a function of the gate voltage, correlated with MIM measurements of the local conductivity (blue) taken at 14 K. Dashed lines are fillings corresponding to the insulating states determined from the MIM measurements. b Zoom-in of the traces from −0.2 V to 3.2 V in a . Full size image Microwave impedance microscopy From Fig. 1c , we extract the PL peak energy position as a function of gate voltage and correlate it with the local conductivity measured through microwave impedance microscopy (MIM) on the same device D1 (see Fig. 2a ). The various dips in the MIM signal indicate the appearance of insulating states whose filling values can be determined by matching its pattern with our prior report [19] . From the MIM data, we identify insulating states at fillings n = 1/4, 1/3, 1/2, 2/3, 3/4, 1, and 2 on the electron side, and n = −1/3, −2/3, and −1 on the hole side. Comparing the MIM with the PL peak position data, we find that most of these fillings also appear in the PL data. The most pronounced ones are the fillings on the electron side, which show blue shifts in the PL peak position. These observed filling values are consistent with recent reports [18] , [19] . Among them, the n = 2 corresponds to the complete filling of the first minibands and the n = ±1 correspond to the Mott insulator states at half filling of these minibands [14] , [15] , [21] . The n = ±1/3, ±2/3, +1/4, and +3/4 correspond to generalized Wigner crystals with a triangular lattice [18] , [19] . The n = 1/2 corresponds to a stripe phase [18] , [19] , [20] . The sensitive readout of the correlated insulating states through the interlayer exciton PL energy can be understood by the larger spatial extent of the interlayer exciton, which renders it more sensitive to the dielectric environment than the intralayer exciton. Similar ideas has been utilized to use the larger 2 s exciton to sensitively probe the correlated insulating states [18] . In addition, the background free nature makes the PL spectra a sensitive probe. At the correlated insulating states, electron interaction results in an energy gap and localizes the electrons, which subsequently modifies the dielectric constant. As a result, both the energy gap seen by the interlayer excitons and their binding energies can be modified, leading to the change in the emission energy, observed as the blueshift of the PL peak at the filling of the correlated states. This picture is consistent with our observation of the larger PL blueshift at n = 1, as the Mott insulator state has a larger gap (~10 meV) compared with other fractional fillings (~2–3 meV) according to previous reports [14] , [15] , [18] , [19] . Power-dependent PL spectra of interlayer excitons The interaction among the interlayer excitons and that between the excitons and the underlying electron solid can be further probed by increasing the interlayer exciton density. 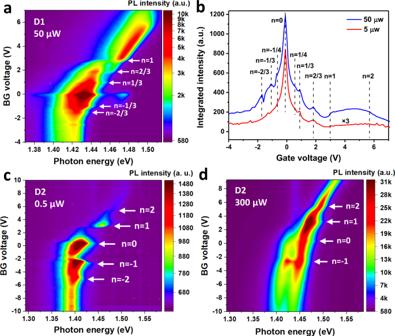Fig. 3: PL of interlayer excitons under increased optical excitation power. aGate-dependent PL spectra of device D1 with the optical excitation power of 50 µW and photon energy centered at 1.959 eV.bIntegrated interlayer exciton PL intensity as a function of gate voltage for device D1 with 50 µW (blue) and 5 µW (red) optical excitation power. Dashed lines are fillings determined from the insulating states from the MIM measurements.c,dGate-dependent PL spectra for device D2 under the optical excitation power of 0.5 and 300 µW. All data are taken at 4.2 K. 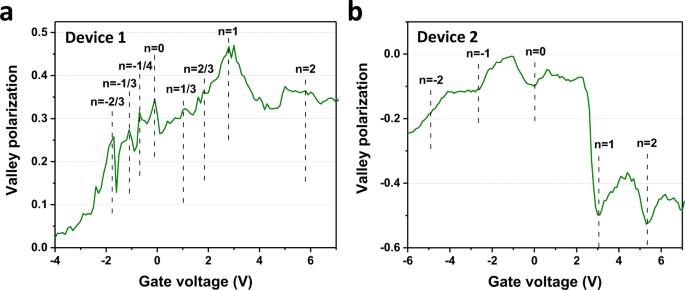Fig. 4: Valley polarization of interlayer excitons in the moiré superlattice. a,bValley polarization for the interlayer excitons in the devices D1 (0° twist angle) and D2 (60° twist angle). The dashed lines are the fillings determined from the MIM measurements. Data are taken at 4.2 K. Figure 3a shows the color plot of the gate-dependent PL spectra of device D1 at an optical excitation power ten times (50 µW) as much as that used in Fig. 1c (5 µW). Compared with Fig. 1c , the higher excitation power data now reveals the states at n = −1/3 and −2/3, which are previously missing in the lower excitation power data. Detailed analysis of the integrated PL intensity as a function of the gate voltage shown in Fig. 3b further reveals the state corresponding to n = −1/4. We perform even more drastic excitation power dependence on another device D2, in which we increase the excitation power from 0.5 µW (Fig. 3c ) to 300 µW (Fig. 3d ). It is obvious that despite the increase of optical excitation by nearly three orders of magnitude, the Mott insulator states at n = ±1 remain intact. This observation is consistent with the picture that the excitons do not destroy the periodic electron solid [4] , [27] . It is worth noting that the asymmetric PL peak shift as a function of the gate voltage for the p - and n -doping sides is due to the difference in the Stark effect related to our specific device structure, which is back gated with the WSe 2 layer closer to the back-gate electrode. Owing to the type-II alignment between WSe 2 and WS 2 , the gate voltage induced holes in the p -doping side will occupy the WSe 2 layer, screening the electrical field between the WSe 2 and WS 2 layer, and reducing the Stark effect. A detailed explanation can be found in Supplementary Note 5 . Fig. 3: PL of interlayer excitons under increased optical excitation power. a Gate-dependent PL spectra of device D1 with the optical excitation power of 50 µW and photon energy centered at 1.959 eV. b Integrated interlayer exciton PL intensity as a function of gate voltage for device D1 with 50 µW (blue) and 5 µW (red) optical excitation power. Dashed lines are fillings determined from the insulating states from the MIM measurements. c , d Gate-dependent PL spectra for device D2 under the optical excitation power of 0.5 and 300 µW. All data are taken at 4.2 K. Full size image One other striking observation is that, in contrast to the intense PL intensity at the charge neutral region ( n = 0) under the low optical excitation power (Fig. 3c ), the PL intensity at the n = 1 state is more strongly enhanced under high excitation power (Fig. 3d ). The time-resolved PL spectra (TRPL) shows a lifetime of 6.5 ns for the n = 1 state (PL peak at ~1.47 eV) and 5.1 ns for the n = 0 state (PL peak at ~1.45 eV) (see Supplementary Note 3 for details). This might arise from the mobility reduction of interlayer excitons at the correlated state at n = 1, in which electrons are localized in the periodic moiré cells. Interlayer excitons can be polarized by the localized charges, inducing an attractive force between the correlated electrons and interlayer excitons that reduces the interlayer exciton mobility compared to the charge neutral scenario ( n = 0). As a result, the chance of nonradiative recombination is reduced, consistent with the TRPL data. It has been shown that the moiré potential can trap interlayer excitons [2] , [4] , [28] , [29] . Our results naturally raise the question of possible localization of interlayer excitons through the additional attraction by the periodic correlated electron solid, which we will explore in future studies. Gate-dependent valley polarization Interlayer excitons also possess valley degree of freedom [30] , which can be probed through helicity-resolved PL spectroscopy measurements. Here we excite both the devices D1 and D2 using the right circularly polarized light ( σ + ) and detect the interlayer exciton PL of the same ( σ + ) or opposite ( σ − ) helicity. The valley polarization \(P\) is calculated by the expression \(P=\frac{I\left({\sigma }^{+}\right)-I({\sigma }^{-})}{I\left({\sigma }^{+}\right)+I({\sigma }^{-})}\) , where \(I\left({\sigma }^{+}\right)\) and I \(\left({\sigma }^{-}\right)\) are interlayer exciton PL intensities with \({{\rm{\sigma }}}^{+}\) and \({{\rm{\sigma }}}^{-}\) helicity, respectively. The valley polarizations as a function of gate voltage for the devices D1 and D2 at 4.2 K are shown in Fig. 4a, b , respectively. The overall valley polarizations for these two devices have different signs due to the different alignment angles (0° for D1 and 60° for D2), and the sign of the valley polarization is consistent with the interlayer exciton at the atomic registry site of \({R}_{h}^{X}\) and \({H}_{h}^{h}\) for the devices D1 and D2, respectively [31] . It is noticeable that the correlated states at both integer and fractional fillings are often associated with an enhanced valley polarization, and the enhancement is most drastic at the fillings of n = 1 and 2 for device D2. This valley polarization enhancement might originate from the decreased valley scatterings due to the interaction between interlayer excitons and correlated electrons. One major valley depolarization mechanism is through Maialle–Silva–Sham mechanism [32] , [33] , which annihilates one exciton in one valley and creates another in the opposite valley. However, when interlayer excitons are attracted by the localized correlated electrons, this probability will likely be significantly suppressed. The correlated electrons, therefore, also provide a tunable platform to manipulate the valleyspin of the interlayer excitons. Fig. 4: Valley polarization of interlayer excitons in the moiré superlattice. a , b Valley polarization for the interlayer excitons in the devices D1 (0° twist angle) and D2 (60° twist angle). The dashed lines are the fillings determined from the MIM measurements. Data are taken at 4.2 K. Full size image Researchers have been inspired to utilize the moiré potential to control interlayer excitons to form an array of quantum emitters. Here we show that the long-range interaction of the electrons in the moiré superlattice can be further exploited for this purpose. The interaction between correlated electrons and interlayer excitons not only allows us to reveal the correlated states at different fillings through the PL spectra, more excitingly, it can be further utilized to control the mobility and valley polarization of the interlayer excitons. Our results, therefore, shed light on how to engineer the interlayer excitons in the TMDCs heterobilayer moiré superlattice for quantum optics and optoelectronics. Heterostructure device fabrication We use a layer-by-layer pickup method to fabricate the WS 2 /WSe 2 heterobilayer device [34] . We first exfoliate monolayer WS 2 , monolayer WSe 2 , few-layer graphene and thin hBN flakes on Si substrate with 285 nm thermal oxide, respectively. We further confirm the crystal orientation of monolayer WSe 2 and WS 2 through second harmonic generation (SHG) measurements (see Supplementary Note 1 for details). We then mount the SiO 2 /Si chip on a rotational stage and use hBN as a stamp to pick up each layer sequentially. The alignment of the monolayer WS 2 and WSe 2 are controlled by fine adjusting the angle of the rotational stage (accuracy of 0.02°) under the microscope, ensuring a near-zero twist angle between the two flakes. The final device is annealed at 140 °C for 6 h in a vacuum chamber. The pre-patterned Au contact electrodes are fabricated through standard electron-beam lithography followed by ebeam evaporation and lift-off processes. Optical characterization The optical measurements are taken with a home-built confocal microscope with spectroscopy capabilities in a liquid helium-controlled optical cryostat. The PL spectra are taken with a CW laser excitation. The reflectance spectra are taken with a supercontinuum white laser source (Fianium). The SHG measurements are taken with a pulsed laser with the width ~160 fs (Ti : Sapphire, Coherent Chameleon). MIM measurements The MIM measurement is performed on a home-built cryogenic scanning probe microscope platform. A small microwave excitation of ~0.1 µW at a fixed frequency around 10 GHz is delivered to a chemically etched tungsten tip mounted on a quartz tuning fork [35] . The reflected signal is analyzed to extract the demodulated output channels, MIM-Im and MIM-Re, which are proportional to the imaginary and real parts of the admittance between the tip and the sample, respectively. The MIM-Im part characterizes the screening of the tip electric field by the sample and changes monotonically with the sample’s local conductivity. Therefore, the dips in the MIM-Im curve plotted in Fig. 2 indicate the appearance of insulating states.